Latent homology and convergent regulatory evolution underlies the repeated emergence of yeasts Convergent evolution is common throughout the tree of life, but the molecular mechanisms causing similar phenotypes to appear repeatedly are obscure. Yeasts have arisen in multiple fungal clades, but the genetic causes and consequences of their evolutionary origins are unknown. Here we show that the potential to develop yeast forms arose early in fungal evolution and became dominant independently in multiple clades, most likely via parallel diversification of Zn-cluster transcription factors, a fungal-specific family involved in regulating yeast–filamentous switches. Our results imply that convergent evolution can happen by the repeated deployment of a conserved genetic toolkit for the same function in distinct clades via regulatory evolution. We suggest that this mechanism might be a common source of evolutionary convergence even at large time scales. Repeated evolution of similar phenotypic traits in distinct clades is common in nature [1] , but the underlying molecular and genomic mechanisms causing similar phenotypes to appear repeatedly are obscure. Among the proposed mechanisms is convergent molecular evolution at the nucleotide or amino-acid sequence level as a result of similar selection pressures [2] , [3] , [4] , [5] . However, parallel changes in coding sequences that lead to functionally equivalent genetic toolkits have an extremely low likelihood and are unlikely to explain the pervasive occurrence of convergence. Yeasts make up a polyphyletic assemblage that originated in multiple distantly related clades of Fungi and include species that spend all or most of their life cycle in a unicellular form [6] , [7] . Species capable of growing as yeasts include some of the most clinically and biotechnologically important fungi and can be found in most major fungal lineages, such as Ascomycota (for example, Saccharomyces cerevisiae, Schizosaccharomyces pombe ) and Basidiomycota ( Cryptococcus neoformans, Malassezia globosa ), but also in earlier diverging (Mucoromycotina) or derived groups, such as the black yeasts in the Pezizomycotina. Importantly, several species with a predominantly yeast-like form can manifest filamentous growth, and several primarily filamentous fungi can grow as yeast under certain conditions (dimorphic fungi) [8] , [9] . The lineages containing unicellular yeast-like species are separated by tens to hundreds of millions of years [10] , but they share remarkable phenotypic and metabolic similarities. To assess the genetic innovations that enabled the convergent evolution of yeasts, as well as the evolutionary consequences of their origins, we compared 59 genomes of filamentous, dimorphic and yeast-forming fungi. We develop a computational pipeline (see Methods) to identify all groups of orthologous genes (orthogroups) and map gene duplications and losses across the organismal phylogeny using Dollo parsimony. We then perform enrichment analyses to identify significantly over- and underrepresented groups among the gene duplications and losses along particular internodes in the phylogeny, and correlate these with evolution of yeast forms using ancestral state reconstruction (see Methods for analytical details). Our results suggest that the potential for yeast growth evolved early in fungal evolution and has been conserved in most groups of fungi. Transitions to yeast-like lifestyle, however, happened much later via changes in the regulatory mechanism of the genetic toolkit for yeast growth, suggesting that the convergent evolution of the yeast phenotype took place via a single origin of the developmental potential followed by convergent changes to its regulation. Inference of genome-wide gene duplication/loss histories We reconstructed the gene duplication and loss history in 59 fungal genomes ( Supplementary Tables 1 and 2 ) using a new computational method that uses Dollo parsimony to map duplications and losses to the organismal phylogenetic tree ( Fig. 1 ; Supplementary Figs 1–3 ). We inferred 286,862 orthogroups, including both multi-species and species-specific (orphan) genes. When species-specific genes (on average, 2–5,000 per species) are excluded, this figure drops to 149,091 orthogroups (51.9%). By mapping the presence/absence of genes in these orthogroups to the organismal phylogeny using Dollo parsimony, we inferred 149,328 gene losses across the 59 species. The resulting gene duplication/loss catalogue ( Supplementary Fig. 1 ) provides information on the gene duplication and loss patterns across the fungal tree, the gene content of common ancestors or genetic innovations along branches leading to the fungal clades included. For instance, we inferred that the last universal common ancestor of fungi had 5,843 gene orthogroups, following a period of high duplication rate and moderate gene loss rate ( Supplementary Fig. 1 ). We used this gene duplication/loss catalogue to identify the evolutionary origins of yeast-like lifestyle and the genomic consequences of transitions to yeast forms in five independently evolved yeast clades. 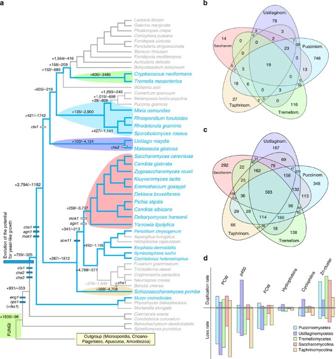Figure 1: Convergent evolution of yeast-like fungi. (a) Reconstruction of the origin of yeast-like growth and the genomic innovations in five major yeast-like lineages (shaded clades). The phylogeny was inferred from a 594-gene partitioned data set, and has maximal ML bootstrap support on all but nine nodes. Highlighted blue path shows the evolutionary origin and phylogenetic distribution of the potential for yeast-like growth. Species in blue are capable of growing as yeast (dimorphic fungi), whereas larger font indicates species spending most of their life cycle in a yeast form. Blue and white bars show the evolution and loss of genes involved in yeast cytokinesis, respectively. Numbers at branches represent duplications (+) and losses (−) inferred by mapping orthogroups onto the species tree by Dollo Parsimony; (b,c) convergence in gene duplications (b) and losses (c) based on PFAM domains and GO terms overrepresented in the five yeast clades. (d) Gene dispensability for genes involved in plant cell wall decomposition (PCW), fungal cell wall biosynthesis and modification (FCW), p450s, hydrophobins, cyclophilins and Zn-cluster TFs. Bars show the rate of gene duplication and loss in the five yeast-like clades, normalized to unit branch length of the tree. Figure 1: Convergent evolution of yeast-like fungi. ( a ) Reconstruction of the origin of yeast-like growth and the genomic innovations in five major yeast-like lineages (shaded clades). The phylogeny was inferred from a 594-gene partitioned data set, and has maximal ML bootstrap support on all but nine nodes. Highlighted blue path shows the evolutionary origin and phylogenetic distribution of the potential for yeast-like growth. Species in blue are capable of growing as yeast (dimorphic fungi), whereas larger font indicates species spending most of their life cycle in a yeast form. Blue and white bars show the evolution and loss of genes involved in yeast cytokinesis, respectively. Numbers at branches represent duplications (+) and losses (−) inferred by mapping orthogroups onto the species tree by Dollo Parsimony; ( b , c ) convergence in gene duplications ( b ) and losses ( c ) based on PFAM domains and GO terms overrepresented in the five yeast clades. ( d ) Gene dispensability for genes involved in plant cell wall decomposition (PCW), fungal cell wall biosynthesis and modification (FCW), p450s, hydrophobins, cyclophilins and Zn-cluster TFs. Bars show the rate of gene duplication and loss in the five yeast-like clades, normalized to unit branch length of the tree. Full size image Reconstruction of the origins of yeast-like growth The origin of yeast-like growth was reconstructed using maximum likelihood (ML) [11] on a collection of 100 species trees sampled from the posterior distribution of a Bayesian Markov chain Monte Carlo phylogenomic analysis [12] comprising 371–594 single-copy genes ( Supplementary Figs 4–5 ). Ancestral state reconstructions placed the origin of the potential for yeast-like growth at the node uniting Mucoromycotina and Dikarya ( Fig. 1 ), which is ~770 million years old [10] . Among the gene duplications inferred for this node, genes related to fungal cell wall biosynthesis, modification and metabolism, including chitin synthases (chitin synthase I, II) and genes with chitin-binding domains (CBM1, CBM5_12, GH18), are significantly enriched ( P =1.89 × 10 −107 –3.54 × 10 −74 , Fisher’s exact test). The orthogroups containing the S. cerevisiae proteins chs2p , chs3p and cts1p , which participate in the build-up and degradation of the primary septum between mother and daughter cells and thus contribute to yeast cytokinesis, originated in this node. Therefore, it is likely that the duplications we observed in this node yielded the paralogues that were adapted for cytokinesis of yeast-like fungi during evolution. Other proteins involved in yeast primary septum synthesis and degradation also appeared early in fungal evolution. Eng1p , an endo-1,3-β-glucanase degrading β-glucans between mother and daughter cells in fission and budding yeast [13] , is a member of a fungal-specific orthogroup that has originated in the node uniting the Entomophthoromycotina, Mucoromycotina and Dikarya, that is, one node before the evolution of yeast-like growth. The origin of the orthogroup containing cps1p (= fks1p, gsc1p ), a cytokinesis glucan synthase previously characterized in fission yeast [14] , budding yeast [15] and Cryptococcus [16] , also localized to this node. The orthogroups containing agn1p (α-glucanase that dissolves the mother cell wall around the septum edge), chs1p (chitin synthase that builds chitin in the primary septum) and mok1p (α-glucan synthase that builds α-glucan in the primary septum) appeared in the node immediately following the evolution of yeast-like growth ( Fig. 1a ). Taken together, these results suggest that the genes involved in yeast cell separation (including the synthesis and degradation of the primary septum) appeared early in fungal evolution in filamentous ancestors and have been conserved throughout the fungal tree. Genes involved in cell division upstream of cell wall degradation (for example, components of the actomyosin ring, septins, Bud proteins [17] ) make up the eukaryotic cell division programme and thus are of more ancient origin (used by unicellular chytrids and microsporidia). Therefore, we suggest that the genetic toolkit for yeast-like growth has been added on top of the eukaryote cell division programme early in fungal evolution and has been widely conserved throughout fungal evolution. This finding explains the widespread occurrence of yeasts and dimorphic fungi with remarkably similar yeast phases among phylogenetically diverse fungal groups. Genomic consequences of the evolution of yeasts Next we examined how yeasts independently became the dominant form in several distantly related clades. We identified orthogroups that originate or show losses in five clades containing predominantly yeast-like forms, including the Saccharomycotina, Taphrinomycotina, Tremellomycetes, part of Pucciniomycetes and Ustilaginomycetes ( Fig. 1a–d ). We inferred minimal genomic innovation (up to 100–636 duplications per clade), but massive gene losses. Functional annotation of the orthogroups that originated in the yeast-like clades revealed little overlap between the genetic innovations inferred for individual clades, suggesting that adaptations of individual yeast clades are mostly lineage specific ( Table 1 ). However, 19 gene ontology (GO) terms and PFAM domains were significantly overrepresented ( P =2.27 × 10 −165 –4.94 × 10 −2 , Fisher’s exact test) among the duplications in all five yeast-like clades ( Supplementary Data 1 ) as well as on the branches leading to the most recent common ancestors of three clades (Saccharomycetales, Taphrinomycotina and Tremellomycetes; Supplementary Table 3 ). We found these GO terms to be significantly overrepresented among duplications in a few other nodes as well, mostly dimorphic fungi and a few others (see Supplementary Information ). All of the 19 GO terms are related to a single transcription factor (TF) family, fungal Zn-cluster TFs (PF00172). Zn-cluster TFs belong to the Zn-finger TF family and regulate a range of processes, including the switches between yeast and filamentous forms in several dimorphic fungi [18] , [19] . Crucially, Ace2 , the principal regulator of cell separation genes Eng1 and Agn1 (ref. 20 ) as well as Mhy1 and Znc1 , which were previously implicated in filamentous/yeast transitions in dimorphic fungi [21] , [22] , also belong to this TF family. Therefore, it is likely that the parallel diversification of this TF family corresponds to the elaboration of the regulatory repertoire governing the maintenance of the unicellular life stage and switches between filamentous and yeast forms. Yeasts maintain a unicellular form through most of their life cycle, whereas their filamentous form is less dominant (as opposed to filamentous and dimorphic fungi) [6] , [8] , [9] . On the basis of the previously reported roles of Zn-cluster TFs, we hypothesize that the expansion of this gene family contributes to the suppression of filamentous forms throughout the life cycle and under different conditions. In support of this, Zn-binding protein families (including Zn-cluster TFs) have been found to have expanded independently in Paracoccidioides immitis also, another dimorphic fungus [23] with a well-developed yeast phase. Table 1 The most important functional gene classes affected by the convergent evolution of yeast clades. Full size table Apart from Zn-cluster TFs, there is hardly any functional gene group undergoing duplications in multiple yeast clades; most innovations are lineage specific (for example, flocculins in Saccharomycotina, Table 1 ). Notably, triglyceride lipases (PF01764) implicated in pathogenicity in both the ascomycete Candida and the basidiomycete Malassezia [24] have independently expanded in the Saccharomycotina (containing, for example, Candida spp. ), Ustilaginomycotina (for example, Malassezia spp.) and Pucciniomycotina ( P <0.01, Fisher’s exact test), although the expansion in the latter yielded a highly divergent subfamily. In contrast to gene duplications, gene losses show high levels of overlap in yeast lineages. We reconstructed 3,000–5,000 gene losses per clade ( Fig. 1a ), for which functional annotation revealed 583 GO terms overrepresented in all five clades and an additional 566 overrepresented in four clades ( Fig. 1b ). Orthogroups showing losses in the five clades are significantly enriched ( P <0.01) for genes related to a range of cellular processes ( Table 1 ), including plant cell wall decomposition, fungal cell wall synthesis and modification, hydrophobins and fungal lysozymes ( Table 1 ). The dispensability of genes involved in cellulose and lignocellulose decomposition, including cytochrome p450 and glutathione-transferase genes, likely reflects the lack of wood-decay capabilities in yeast-like fungi [6] . Further, our results indicate that transitions to yeast-like lifestyle induce a complete loss of hydrophobins (except in Ustilaginomycetes), which confer hydrophobicity to cell surfaces, and have been implicated in switching between aqueous and aerial phases of hyphae and fruiting body development [25] . As expected, gene classes significantly underrepresented among the losses (that is, non-dispensable) include those required for essential cellular processes, such as DNA replication, sequence recognition, chromatin binding, chromosome segregation (see Supplementary Data ). Notably, TFs, as well as intra- and extracellular transport-related genes, do not show extensive losses and appear indispensable for yeasts, which might reflect conservation of genes involved in multicellular growth and foraging abilities. The observed pattern of parallel deployment of the genetic toolkit of yeast-like growth in distantly related clades via independent changes in its regulatory mechanism is inconsistent with classical models of convergent evolution [1] , [3] , [26] , [27] . Our study suggests that this mechanism can generate signatures of convergent evolution at the phenotype level, while the underlying effector genes evolved only once and remained unexpressed with regard to the phenotype (possibly involved in other processes). Rather, convergence was observed in their regulation, which resulted in repeated emergence of yeast-like development as the dominant phase of the life cycle in phylogenetically distant clades ( Fig. 2 ). It has been proposed that latent homologies [28] , [29] , [30] (for example, developmental modules, regulatory circuits or genes) can underlie the repeated origins of similar traits in distant clades if they can easily be recruited for the same new functionality. Such latent homologies should, however, be under selection to be maintained over vast time scales, in this case, hundreds of millions of years. Therefore, we hypothesize that structures underlying such latent homologies are pleiotropic (explaining their maintenance) and that simple changes in their regulation can lead to their repeated deployment for the same new function in different clades. Latent homologies may thus explain the repeated appearance of similarity by predisposing lineages for evolving certain phenotypes, without the need for parallel evolution of equivalent genetic toolkits and might be a common source of convergence in complex phenotypic traits throughout the tree of life. 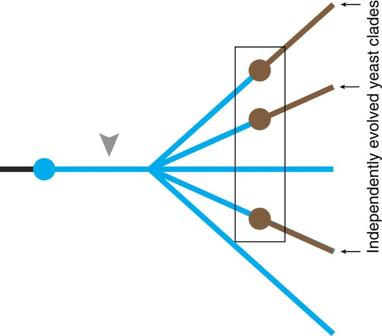Figure 2: Schematic model of the mechanism proposed here. The genetic toolkit of yeast-like growth (blue circle) evolved early but remained latent (possibly involved in different functionalities). Subsequently, the genetic toolkit has been deployed for new functions via simple changes in their regulation (black rectangle). Figure 2: Schematic model of the mechanism proposed here. The genetic toolkit of yeast-like growth (blue circle) evolved early but remained latent (possibly involved in different functionalities). Subsequently, the genetic toolkit has been deployed for new functions via simple changes in their regulation (black rectangle). Full size image Overview of the COMPARE strategy COMPARE (comparative phylogenomic analysis of trait evolution) is designed to make inferences about the genetic background of a trait based on whole-genome sequence data and phylogenetic correlation ( Supplementary Fig. 2 ). It achieves that by reconstructing the gene duplication and loss history in the input genomes in relation to the phenotypic trait of interest and filtering orthogroups evolving in a correlated fashion with the trait. Such orthogroups are expected to include the ones participating in the development of the trait, thus COMPARE can unravel the genetic background of a phenotypic trait in the absence of extensive transcriptomics resources or mechanistic data. The pipeline can be run on multiple whole genomes or a subset of gene families. The analytical core of COMPARE, orthologue coding ( Supplementary Fig. 3 ), improves on previous methods for resolving orthology and paralogy by identifying orthogroups based on reconciled ML gene trees and explicitly distinguishing duplications from speciation events. COMPARE performs well on large multi-gene families with intricate duplication and loss history (shown by simulation studies, unpublished results). Previous approaches to the same problem identified orthogroups on the basis of reciprocal best BLAST hits or genetic distances, which do not explicitly model duplication and speciation events, thereby falling short in capturing patterns of vertical inheritance of functionality through speciation versus the opportunity for neo- or subfunctionalizations following duplication events [31] , [32] . Protein clustering, alignment and gene tree inference We clustered predicted protein sequences in the input genomes based on similarity using the MCL algorithm [33] with an empirically determined inflation parameter of 2.0. The clustering used JGI’s pipeline. Clustering of a total of 614,942 proteins in the 59 input genomes resulted in 225,476 clusters with an average size of 9.28 proteins per cluster (singletons excluded). The largest cluster contained 1,912 protein sequences, while there were 178,440 clusters made up of a single protein only. We subjected these to BLAST searches against the non-redundant protein database in NCBI. As a conservative way of accounting for potential gene prediction errors, we excluded from the further analyses all proteins that show no similarity to any other protein sequence (self-hits were not considered) in the NCBI database. It is likely that by this strict criterion, we excluded some accurately predicted proteins as well, however, this is unlikely to affect our results, since single-species-specific proteins played an insignificant role in our analyses. MCL clusters have been shown to correspond well to gene families [33] , so hereafter we use cluster and gene family interchangeably. Although MCL has been shown to achieve high accuracy in reconstructing gene families, the delimitation of gene families on the basis of similarity only is challenging and depends among others on the (subjective) choice of inflation parameter. The crucial aspect of clustering for COMPARE is to infer monophyletic groups of proteins in the same clusters—whether these clusters accurately represent gene families or not is of secondary importance, since clusters will be split into orthogroups, which form the basis of subsequent steps of the analyses. Subsequently, a multiple sequence alignment was estimated for each cluster by using PRANK v.111130 (ref. 34) [34] with default settings and the ‘+F’ option switched off. For each sequence alignment, ML gene trees were then estimated in RAxML 7.2.8 (ref. 35 ) under the PROTGAMMAWAG model for clusters smaller than 50 proteins or the PROTCATWAG for clusters >50 proteins. RAxML was launched with default settings. Since gene trees are known as a potential source of error in genomic studies and the topology can significantly influence downstream steps of the analysis, we incorporated a gene tree improvement step into the pipeline. We used TreeFix [36] , a gene tree–species tree reconciliation algorithm that performs topological changes on the gene tree and searches for alternative topologies that minimize the duplication/loss cost while having a likelihood statistically not significantly worse than that of the ML topology. TreeFix was run with the default reconciliation model (duplication/loss cost) and RAxML as the estimator of site-wise likelihoods. We allowed rerooting of the input gene trees if it decreased the duplication cost. P values were obtained by the Shimodaira–Hasegawa test [37] and a 0.05 cutoff was applied. Aligned sequence data for organismal phylogenies and Supplementary Data 1 are available at DRYAD ( http://dx.doi.org/10.5061/dryad.4rp68 ). Orthologue coding and the reconstruction of duplication-loss histories In the core of the COMPARE pipeline lies orthologue coding ( Supplementary Fig. 3 ), the algorithm that identifies sets of orthologous genes in gene trees and codes them into an orthologue presence/absence matrix. By using reconciled gene trees computed from gene family alignments, orthologue coding is expected to be more accurate in finding orthologous groups than any previous method. The algorithm takes a (reconciled) gene tree as input and first scores each node of the gene tree either as a duplication or a speciation node, based on taxon overlaps between its descendent subtrees. Then, it identifies the most inclusive path on the gene tree that contains only one gene per species and that does not include more than one subtree of duplication nodes, but all subtrees of speciation nodes. A set of orthologous genes delimited this way is assigned to an orthogroup and coded as a presence/absence character where species having the orthologue are assigned a ‘1,’ whereas species lacking it are assigned a ‘0’. The path connecting proteins in the first orthogroup is then deleted from the gene tree, resulting in multiple subtrees; the algorithm iterates over all subtrees until all the terminals in the gene tree have been assigned to an orthogroup. Note that at this step, the internal relationships within the orthogroup are not required to be consistent with the species relationships. The collection of binary characters representing all the closest orthologous sets found in a gene tree is saved into a matrix, which in the current implementation is a NEXUS formatted file [38] . Importantly, the NEXUS file stores (as comments) two types of information associated with each orthogroup: first, the protein IDs of the terminals, which make up the orthogroup, and the list of taxa found in the sister clade of the subtree in which the path connecting proteins in the orthogroup originated. This latter is crucial for reconstructing the point of duplication in the species tree that gave rise to the orthogroup, since the node in which the duplication happened is the least inclusive subtree containing the species defined by the union of the taxa in the orthogroup and its sister clade. A flowchart illustrating the orthologue-coding algorithm is presented in Supplementary Fig. 2 . Orthologue coding as described above is applicable to gene trees. However, there are gene families that contain less than four proteins, among which the evolutionary relationships are described by a star tree (three proteins) or cannot be represented as a tree structure at all (two and one protein families). Inference of orthology/paralogy relationships in these cases used a simplified (but logically nested) version of the orthologue coding algorithm. We designated as an orthogroup the most inclusive set of proteins in the gene family that contains only one protein per species. Orthogroups coded this way were added to the binary presence/absence matrix. Of gene families smaller than four proteins, we only considered those that either contained proteins from multiple species or showed significant sequence-level similarity (as inferred by BLAST on NCBI) to a protein known from a different species. By this criterion, we excluded a large number of potential annotation and prediction errors, which would have otherwise added noise to our analyses. Following orthologue coding, we reconstructed the duplication/loss history for each orthogroup across the input genomes on the species tree by using Dollo parsimony [39] , [40] , [41] , which allows one gain and any number of losses per orthogroup on the species tree. We mapped orthogroups coded from one gene tree at a time and recorded the number of gains (duplications) and losses along each branch of the species tree ( Supplementary Fig. 1 ). Gene tree error can have a profound effect on the inference of duplication and especially loss events in gene tree–species tree reconciliation methods [36] . Because COMPARE uses gene trees to identify closest orthologous groups and indirectly to reconstruct the duplication/loss history in the input genomes, it might also be prone to this source of error. One way to account for this in our pipeline is to reconcile the gene trees with the species tree using TreeFix, which has recently been shown to dramatically improve the accuracy of duplication/loss inference over purely sequence-based trees [36] . To further examine the robustness of our results to input gene tree quality, we performed a mapping on three gene tree collections, of which one was the set of gene trees reconciled by TreeFix, another was the purely sequence-based ML trees (from RAxML) and the third was midpoint-rooted ML trees. We found that the number of inferred duplications were relatively robust, whereas the number of losses differed more significantly between the three mappings. However, the general trends of duplications/losses across the tree were unaffected, including the outstanding numbers of losses on the branches, leading to the five predominantly yeast-like clades. Therefore, we conclude that the extensive convergent gene losses we observed in these clades are not affected by gene tree error. COMPARE is implemented in Perl and is available from the authors. The gene duplications/loss catalogue describing genome evolution in the 59 genomes (including reconstructed orthogroups and Dollo parsimony mapping), protein clustering, gene family alignments and reconciled gene trees, as well as custom scripts and programme code, are available from the authors on request. Taxon sampling We sampled 59 genomes representing all major sequenced lineages of Fungi and a collection of outgroup species. We included 24 species of yeasts or dimorphic fungi that can grow as yeasts under certain conditions. To support the inference of gene duplication/loss events in early evolution Fungi, we included a set of outgroup taxa from lineages closely related to fungi, including Microsporidia ( Trachipleistophora hominis , Encephalitozoon cuniculi and Antonospora locustae ), Choanoflagellata ( Monosiga brevicollis , Salpingloea rozetta ), Apusozoa ( Thecamonas trahens ) as well as Amoebozoa ( Dictyostelium discoideum and Entamoeba histolytica ), to root the tree. Within fungi, we included representatives of the earliest diverging lineages Kickxellomycotina ( Coemansia erecta ), Entomophthoramycotina ( Conidiobolus coronatus ), Chytridiomycota ( Batrachochytrium dendrobatidis and Spizellomyces punctatus ), as well as representatives from the Mucoromycotina (3 spp. ), Ascomycota (23 spp.) and Basidiomycota (22 spp. ; Supplementary Table 1 ). All lineages of sequenced yeast-like fungi are represented in the data set, including species that grow exclusively as a unicellular yeast form, as well as dimorphic fungi, which can switch between hyphal and unicellular forms. The data set contains both basidiomycetous and ascomycetous yeasts, including the representatives of the budding and fission yeasts. Ascomycetous black yeasts are represented by Exophiala dermatitidis ( Wangiella dermatitidis ). A wide range of ecological strategies is also covered, including opportunistic human-, animal- and plant pathogens, free-living saprobes, rock-dwelling black yeasts, as well as intracellular parasites ( Mixia osmundae [42] ). The distribution of fungi capable of growing as yeast are shown in Fig. 1 and Supplementary Table 2 . Organismal phylogenetic analyses We inferred a species tree based on single-copy genes by ML and Bayesian Markov chain Monte Carlo. We identified single-copy gene families among the MCL clusters (inflation parameter: 2.0), which were represented in at least 15 species, as well as ones that were not strictly single copy, but in which duplications happened only on terminal branches (that is, only inparalogues were allowed). Gene families with deep paralogues (based on ML gene trees) were excluded. In the case of gene families showing terminal duplications only, we chose one of the inparalogues randomly for phylogenetic analyses, the rest were not considered further. Single-gene alignments were inferred using PRANK v.111130 (ref. 34) [34] with default settings, one round of alignment improvement and invoking the option to output XML formatted alignment files in addition to fasta. Gene trees were inferred in RAxML 7.2.8 (ref. 35) [35] under the GTRGAMMA model of evolution. Single-gene alignments were further filtered for potential non-orthologous sequences (following ref. 43 ) and incongruent phylogenetic signal by comparing weighted Robinson–Foulds distances [44] across all pairwise comparisons. We excluded ambiguously aligned and low-reliability region from the alignments by inspecting site posterior probabilities calculated by PRANK and stored in the XML files. For each alignment site, we summed the posterior probabilities over all residues and calculated their mean; only sites for which the mean of the posterior probabilities exceeded a pre-set threshold were retained. These analyses were done using a custom-written Perl script (FilterPostProb.pl), which is available from the authors upon request. We used three different thresholds: 0.95, 0.98 and 1.0. A threshold of 1.0 means that only alignment columns for which all residues have a posterior probability of 1 are retained for phylogenetic analyses. This represents a very strict criterion, yet missing sequences are not counted as gaps (unlike in GBlocks), which means that even if some species lack sequence data for that gene, alignment accuracy will be evaluated in the context of the species that have sequence. Furthermore, since PRANK posterior probabilities take into account the insertion–deletion process, high-reliability regions with indels will be retained. Single-gene alignments longer than 50 amino acids were concatenated into a supermatrix, with recording the start and end positions of input alignments for setting up partitioned models. We obtained three data sets, corresponding to the three different thresholds of site exclusion, 0.95, 0.98 and 1.0. These included 171,073–51,789 amino acids and 594–371 gene families ( Supplementary Table 3 ). Taxon occupancy was very homogeneous across the taxa (on average, 71% of all the loci per species), with the exception of Microsporidia, which were represented by significantly fewer loci than the average (~14%), however, this did not seem to affect the placement of Microsporidia, its inferred position was congruent with that inferred in previous studies. We performed ML and Bayesian phylogenetic inference using both partitioned and unpartitioned models. During initial runs, we considered the data sets as a single partition, but in subsequent analyses the data sets were partitioned into single-gene alignments and the model parameters were estimated separately. The tree topology obtained in partitioned and unpartitioned runs were identical; however, we preferred partitioned models, which have been shown to outperform unpartitioned ones in several previous benchmarks [45] , [46] , [47] , [48] . Bayesian phylogenetic analyses were performed in Phylobayes 3.3 (ref. 12) [12] . We ran three replicates with one chain per replicate and a chain length of 100,000 cycles. The CAT mixture model of protein evolution was used [49] . Burn-in values were established by checking convergence in likelihood values and clade posterior probabilities by using AWTY [50] . The trees from three independent runs remaining after the exclusion of burn-in were summarized in a 50% majority rule consensus tree by using the Sumtrees.py script of the Dendropy package [51] . Results of the Bayesian phylogenomic analyses are shown in Supplementary Fig. 5 . For all data sets, ML bootstrapping was performed using the PTHREADS version of RAxML 7.2.8 (ref. 35 ). We ran 1,000 thorough bootstrap replicates for each data set, using the rapid hill climbing algorithm and a partitioned model. Bootstrapped trees were summarized and mapped to the ML tree using the SumTrees script of the Dendropy package [51] . The ML trees from two data sets (threshold 0.98 and 1.0) were identical to each other and congruent with our current understanding of the relationships between these taxa, whereas the data set with the least stringent criteria for data exclusion (threshold 0.95) placed Microsporidia in a clade together with Entamoeba histolytica and left the Amoebozoa polyphyletic ( Supplementary Figs 4 and 5 ). However, this data set had the largest concatenated length (171 kb) with the fewest ambiguously aligned and fast-evolving sites removed, which is likely to have caused the unexpected placement of Microsporidia. The difficulty of resolving the phylogenetic placement of this clade is well documented in the literature [52] , [53] , [54] , and is mostly caused by the high rate of molecular evolution of their genomes. In the light of this, it is not surprising that out of our three data sets, the one with the least stringent criterion for data inclusion (and thus likely more noise) showed the highest uncertainty in the placement of this clade, whereas two out of three with more stringent criteria inferred a placement that is in agreement with previous multi-locus and phylogenomic studies. We observed some uncertainty in the support values of nodes adjacent to Microsporidia, namely, in the placement of choanoflagellates and Thecamonas ; however, despite the somewhat lower support values, the topology of the trees is identical to previously published phylogenies. Apart from the unexpected placement of Microsporidia in the least stringent data set, the ML bootstrap analyses provided strong support at nearly every node of the phylogeny. Weaker support (51–73%) was observed for the placement of the Pucciniomycetes relative to the Ustilaginomycetes, a node that has been known as difficult to resolve in the Basidiomycetes [55] . We performed ancestral character state reconstructions on a Bayesian tree sample obtained from the posterior distribution of the PhyloBayes analyses. We coded each species as capable of growing as yeast or not according to Supplementary Table 2 (that is, only the potential was scored, not considering how much of the lifestyle the fungus spends as a yeast form). We used the ML method as implemented in BayesTraits 1.0 (ref. 56 ) with 50 ML attempts per tree. Model parameters were estimated by the programme. We used the ‘addmrca’ command to define nodes for which ancestral states were reconstructed. A difference of two log-likelihood units was considered strong support for the better fitting state. Enrichment analyses From the global mapping across the 59 genomes, we extracted for each of the five yeast-like clades the orthogroups that originated or showed a loss in that clade. We prepared two versions of these lists, one in which only the orthogroups showing a change (duplication or loss) on the branch leading to the clade are included and one in which orthogroups gained or lost on any of the branches within that clade were included (see Supplementary Data 1 ; labelled as ‘node’ and ‘subtree’, respectively). In other words, one version focused on the events that happened only on the branch leading to the clade, whereas the other considered all duplications and losses inferred in that clade. Further, of the latter whole-clade lists we prepared two versions, one that contained all orthogroups and another that excluded single-species-specific orthogroups (orphan genes, labelled as ‘inparalogues’). The reason for excluding proteins known from only one species is that these often do not have detectable PFAM domains, are partial genes or otherwise questionable predictions, potentially introducing error into the analyses. This approach yielded 3 lists of orthogroups gained and 2 lists of orthogroups showing loss(es) for a single clade (except for Schizosaccharomyces , a single-species clade for which two and one lists were obtained, respectively), resulting in 14 lists of gains and 9 of losses altogether. These lists were used to determine the functional gene categories and PFAM domains that show more duplications or losses than expected by chance in each of the five clades. Proteins were annotated using the PFAM database version 22 (ref. 57 ). PFAM domains were subsequently mapped to GO terms [58] . We also examined whether Zn-cluster TFs show significant overrepresentation among the duplications in parts of the tree other than the five yeast clades. For this, we prepared lists of orthogroups showing duplications in each of the nodes in the phylogenetic tree (119 nodes) and performed enrichment analyses as described above. These analyses revealed overrepresentation of Zn-cluster TFs among the duplications in the same yeast-like clades plus those of some additional nodes ( E. dermatitidis , Symbiotaphrina kochii , Cochliobolus heterostrophus , Penicillium chrysogenum , Fusarium graminis , Fomitiporia mediterranea , Wallemia sebi and the node connecting Exophiala and Symbiotaphrina , the one connecting Penicillium , Aspergillus and Histoplasma ). Many of these species are dimorphic (see Fig. 1 ) with a more or less developed yeast phase in their lifestyle, so the expansion of Zn-cluster TFs in these taxa is consistent with our hypothesis. Their expansion in non-dimorphic fungi ( Fusarium , Fomitiporia , Wallemia , Aspergillus ), however, likely corresponds to the recruitment of this TF family for other functions. Custom scripts were developed in Python and R to analyse over- and underrepresentation of functional annotation terms in orthogroups using the Fisher Exact test. The Benjamini–Hochberg correction was used to correct for multiple testing using a P value of 0.05. How to cite this article: Nagy, L. G. et al. Latent homology and convergent regulatory evolution underlies the repeated emergence of yeasts. Nat. Commun. 5:4471 doi: 10.1038/ncomms5471 (2014).